Ultra-low-loss optical delay line on a silicon chip Light propagation through an optical fibre causes a long, non-resonant (true) time delay used in numerous applications. In contrast to how it is deployed in optical communication systems, fibre is coiled in these applications to reduce footprint. This is a configuration better suited for a chip-based waveguide that would improve shock resistance, and afford the possibility of integration for system-on-a-chip functionality. However, integrated waveguide attenuation rates lag far behind the corresponding rates of optical fibre, featuring attenuation many orders larger. Here we demonstrate a monolithic waveguide as long as 27 m (39 m optical path length), and featuring broadband loss rate values of (0.08±0.01) dB m −1 measured over 7 m by optical backscatter. Resonator measurements show a further reduction of loss to 0.037 dB m −1 , close to that of optical fibres when first considered a viable technology. Scaling this waveguide to integrated spans exceeding 250 m and attenuation rates below 0.01 dB m −1 is discussed. Fibre-optic waveguides for true time delay are used in rotation sensing, radio frequency photonics, high-stability microwave oscillators and all-optical signal processing [1] , [2] , [3] , [4] , [5] , [6] , [7] . Transfer of these applications to a wafer imposes new challenges on microphotonic fabrication. Waveguide loss must be reduced to unprecedented, low levels and maintained over a broadband spectral region. Also, the process must scale so as to maintain these low-loss levels in a continuous waveguide structure over broad areas. Concerning waveguide loss, the lowest attenuation rates are obtained for a silica-based or silica-clad guide, and there has been interest in the practical limits of optical loss in such structures [8] , [9] , [10] . For a pure silica core waveguide [10] the state-of-the-art does not reflect fundamental material limits, but is instead set by interface roughness on the waveguide itself. Certain processes can heal out this roughness. Laser-induced reflow of thermal silica has been used to create ultra-high-Q toroidal-shaped resonators [11] , but comparably low attenuation rates have not been possible in adapting this technique for waveguide fabrication [12] . Likewise, thermal reflow is possible by introducing dopants such as phosphor and boron so as to lower the melting point of silica below that of silicon. However, the doping process has been observed to increase material optical loss [13] . Characterization of attenuation rate in a very-low-loss integrated waveguides is complicated by the insertion loss associated with coupling light into the guide. The most reliable characterization methods avoid this problem entirely by using either resonators or optical backscatter reflectometry. Resonator Q measurements have long been recognized as a reliable way to characterize spans of waveguide configured into closed-loop whispering galleries [8] , because the Q-factor in the under-coupled limit depends only on waveguide attenuation. Although this method is an accurate way to test loss over a small area, the ultimate goal of replacing optical fibre in certain applications requires much greater spans of waveguide than has been typical in photonics. Local testing of either short spans of waveguide or resonators, while important, is not a sufficient test of device uniformity or fabrication scalability. Over large length spans, optical backscatter reflectometry provides attenuation versus propagation distance that captures attenuation variability caused by wafer-scale variation of the fabrication process [14] . Using backscatter reflectometry, an integrated silica waveguide (length 10 m) with loss of 1.7 dB m −1 and a silicon nitride in silica guide (length 6 m) with loss of 2.9 dB m −1 have been demonstrated [9] , [10] . Moreover, a silicon nitride waveguide configured into resonators has produced even better results around 1.1 dB m −1 (ref. 15 ). A loss of 0.3 dB m −1 has been reported for a silica guide [16] ; and recently, loss less than 0.1 dB m −1 at 1,580 nm (rising to 0.8 dB m −1 at 1,540 nm) has been reported for a 1-m long silicon nitride waveguide using a backscatter method [17] . Beyond achieving very low optical loss values, long delay lines present a new and non-trivial device challenge with respect to optical micro-fabrication. The combination of the large field size, susceptibility to single-point failure and required low transmission loss, make them sensitive to process-induced defects and defect density levels that might otherwise be tolerated in smaller-area, higher-loss devices. The fabrication process demonstrated here uses only conventional techniques. Specifically, only conventional lithography as well as wet and dry etching are performed. This enables visible defects and voids to be maintained at levels no greater than unity over areas of 50 cm 2 , ensuring no breaks in transmission. This is an advantage over techniques such as wafer bonding [18] . In this study, both optical backscatter reflectometry and resonator Q measurements are used to confirm waveguide loss. Average measured waveguide loss of 0.08±0.01 dB m −1 in long spirals is inferred from backscatter measurements over a broad band of wavelengths in the telecommunications window. Also, narrow-band backscatter measurements are used to study the wavelength dependence of the loss and a lower limit of 0.05±0.015 dB m −1 is measured. Moreover, a lower value of 0.037 dB m −1 is obtained with resonator-based measurements. As a simple application of these new devices, a data stream is also transmitted through a delay line to illustrate a data buffer function. The waveguide delay lines reported are the longest, ultra-low-loss devices demonstrated to date and the ultra-low-loss window is shown to be broadband, spanning the telecommunications window. Moreover, by showing that fields containing long sections of waveguide can be stitched to create an even longer continuous waveguide, the approach is shown to be scalable. Structures over areas as large as 9.5 cm×9.5 cm are demonstrated and delays as long as 250 m are feasible. Fabrication process and waveguide structure To fabricate the waveguide delay line, we have adapted a technique for realization of high-Q silica whispering-gallery resonators. Therein, disk resonators with Q factors as high as 50 million (0.5 dB m −1 ) have previously been demonstrated using lithography, followed by a buffered HF etch and XeF 2 dry etch of the silicon [19] . In those devices, a distinctive wedge profile was applied to isolate the optical mode from the rough lithographic edge. By creating a small-angle wedge, the mode was pushed away from the edge, thereby lowering scattering loss and boosting Q factor. After careful study of this process, we have found that proper etch control can eliminate the lithographic roughness altogether. As illustrated in Fig. 1 , two competing etch fronts regulate whether the roughness is present. By allowing the etch time to run longer, a single etch front results and ultra-low-loss structures can be fabricated over a wide range of angles (8–30°). A long waveguide based on this wedge geometry was prepared in the form of an Archimedean whispering-gallery spiral. A cross-section is shown in Fig. 1 . In the current design, only one edge of the oxide is used for waveguiding. As discussed later, a ridge design can enable use of the inner edge thereby boosting the areal efficiency of the delay structure. Finally, oxide thickness was increased from previous work so as to further reduce surface scattering loss. A thickness of 8 μm was used in the present devices. 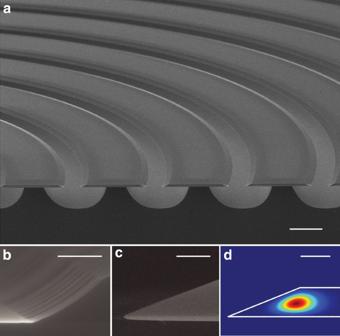Figure 1: An SEM micrograph showing a cross-section of the spiral delay line. (a) Silicon pillars support thermal oxide structures, the outer edge of which guides the optical mode. (b) Close-up view of oxide edge that is formed using a non-optimized etch. Two etch fronts are apparent along with roughening of the oxide surface. (c) Close-up view of oxide edge that is formed using an optimized etch. Etch duration has been increased to eliminate one of the etch fronts, resulting in a smooth edge. (d) The finite element simulation of the fundamental optical mode propagating inside the waveguide. Scale bars: (a) 100 μm; (b) 0.5 μm; (c) 0.5 μm; (d) 8 μm. Figure 1: An SEM micrograph showing a cross-section of the spiral delay line. ( a ) Silicon pillars support thermal oxide structures, the outer edge of which guides the optical mode. ( b ) Close-up view of oxide edge that is formed using a non-optimized etch. Two etch fronts are apparent along with roughening of the oxide surface. ( c ) Close-up view of oxide edge that is formed using an optimized etch. Etch duration has been increased to eliminate one of the etch fronts, resulting in a smooth edge. ( d ) The finite element simulation of the fundamental optical mode propagating inside the waveguide. Scale bars: ( a ) 100 μm; ( b ) 0.5 μm; ( c ) 0.5 μm; ( d ) 8 μm. Full size image Backscatter characterization of single-spiral delay lines An optical backscatter reflectometer (Luna OBR 4400) was used to characterize each delay line. 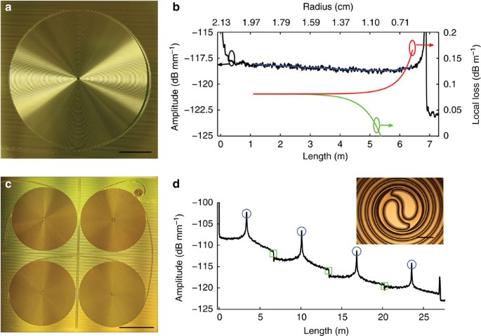Figure 2: Optical micrographs and backscatter reflectometer data for a single spiral and a monolithic spiral cascade. (a) An optical micrograph of a 7-m physical path length, counter-clockwise spiral. This spiral has a diameter of 4.3 cm. (b) Optical backscatter reflectometer measurement of the spiral waveguide shown ina. On account of the return path, the backscatter decay rate is increased twofold. The blue curve is a fit to the backscatter level, while the green curve gives a fit to the local backscatter decay rate and the red curve uses a model to infer the actual local waveguide attenuation, which is approximately 0.08 dB m−1over most of the spiral. The upper axis gives the radius from centre, while the lower axis gives the physical path length. (c) Optical micrograph of a cascaded, four-spiral waveguide having a physical path length of 27 m. The input port is in the upper left of the image, and the waveguides connecting neighbouring spiral delays are visible. The entire chip is 9.5 cm×9.5 cm and consists of four, separately exposed and stitched lithography fields. (d) Optical backscatter reflectometer measurement of the spiral waveguide delay line shown inc. The periodic singularities (blue circles) in the backscatter signal correspond to the optical wave transiting the inner adiabatic coupling region of each spiral. Other discontinuities (green squares) in backscatter occur when the optical wave transfers between the spirals and result from higher-order transverse modes being mode filtered. The inset todis a magnified view of the adiabatic coupling section, which is approximately 1 mm in diameter. Scale bars: (a) 1 cm; (c) 2 cm; (d) 500 μm. Figure 2a shows a spiral with a path length of approximately 7 m. (All path lengths quoted here are physical path lengths, and optical path lengths are about 1.45 times longer.) The cleaved facet input is at the lower left corner of the chip and features a 7° cleave angle so as to reduce Fresnel reflection for backscatter reflectometer measurements. Optical fibre and index-matching oil are used for coupling. The waveguide is a single, counter-clockwise Archimedean spiral that terminates near the centre of the spiral. As noted in Fig. 1 , waveguiding occurs on the outer edge of the silica. The undercut to the silica must therefore be sufficient to eliminate scattering of the fundamental guided mode with the silicon pillar. Both calculation and measurement (see discussion of Fig. 2c ) show that an undercut of 60 μm is sufficient to lower this silicon pillar interaction to levels below that caused by silica surface scattering. In backscatter measurements, however, the presence of a few higher-order radial modes will produce an enhanced backscatter signal due to their stronger interaction with the silicon pillar. For the same reason, these modes also show higher waveguide attenuation, masking the underlying fundamental-mode optical loss. To prevent this masking effect, the undercut in Fig. 2a has been increased somewhat beyond what is necessary for the fundamental mode. By doing this, even higher-order radial modes excited by the input fibre will experience a negligible level of pillar scattering. This behaviour is observed by monitoring backscatter signal in spirals of increasing undercut. The backscatter decay rate is observed to steadily decrease and finally plateau at around 75 μm of undercut. Figure 2: Optical micrographs and backscatter reflectometer data for a single spiral and a monolithic spiral cascade. ( a ) An optical micrograph of a 7-m physical path length, counter-clockwise spiral. This spiral has a diameter of 4.3 cm. ( b ) Optical backscatter reflectometer measurement of the spiral waveguide shown in a . On account of the return path, the backscatter decay rate is increased twofold. The blue curve is a fit to the backscatter level, while the green curve gives a fit to the local backscatter decay rate and the red curve uses a model to infer the actual local waveguide attenuation, which is approximately 0.08 dB m −1 over most of the spiral. The upper axis gives the radius from centre, while the lower axis gives the physical path length. ( c ) Optical micrograph of a cascaded, four-spiral waveguide having a physical path length of 27 m. The input port is in the upper left of the image, and the waveguides connecting neighbouring spiral delays are visible. The entire chip is 9.5 cm×9.5 cm and consists of four, separately exposed and stitched lithography fields. ( d ) Optical backscatter reflectometer measurement of the spiral waveguide delay line shown in c . The periodic singularities (blue circles) in the backscatter signal correspond to the optical wave transiting the inner adiabatic coupling region of each spiral. Other discontinuities (green squares) in backscatter occur when the optical wave transfers between the spirals and result from higher-order transverse modes being mode filtered. The inset to d is a magnified view of the adiabatic coupling section, which is approximately 1 mm in diameter. Scale bars: ( a ) 1 cm; ( c ) 2 cm; ( d ) 500 μm. Full size image Backscatter data in Fig. 2b are obtained for such a deeper undercut spiral. With the exception of the narrow-band spectral study in Fig. 5 , all backscatter data are taken using a broadband setting (approximately 90 nm span in the 1,550 nm band) [14] . The data show a linear decrease (on the log scale) over nearly the full 7 m of the spiral path. The inferred loss rate from this data is 0.05±0.01 dB m −1 and provides a lower bound on the waveguide attenuation rate. This value accounts for the optical return, which increases the observed backscatter attenuation rate by twofold. To further refine the estimate, the impact of the varying backscatter signal caused by the changing radius of curvature is accounted for in the measurement. For this calibration, we first note that bending loss data in Fig. 3, when compared with attenuation calculation based on atomic force microscope (AFM) roughness data, show that surface roughness scattering is the principle source of attenuation to diameters at least as large as about 1 cm. By assuming that backscatter strength is proportional to attenuation, a simple differential equation relates the measured backscatter power, B ( z ), to local waveguide attenuation, α ( z ). The equation is given by, This equation shows that when the attenuation rate is changing with distance (in the present case on account of the slowly changing radius of the waveguide), there is a slight correction to the loss as inferred from the backscatter rate. Inward spiraling waves produce a backscatter signal that attenuates more slowly on account of this term, while outward spiraling waves appear to decay more quickly. By using the measured backscatter data as input to the above equation, a corrected value of 0.08±0.01 dB m −1 for the loss of the device, in Fig. 2a, is obtained. Figure 5: The wavelength dependence of waveguide loss. The loss is measured with backscatter reflectometry over a wavelength range of 1,528 to 1,608 nm in a 7-m long spiral waveguide. 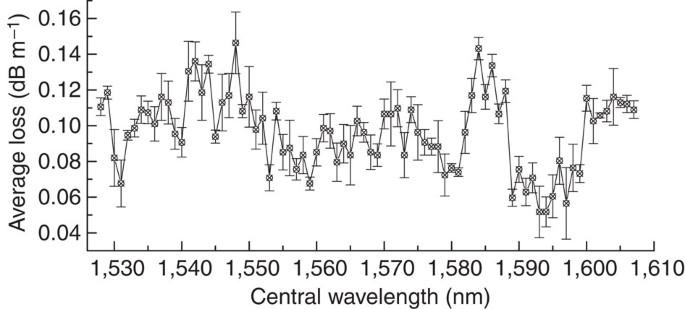Figure 5: The wavelength dependence of waveguide loss. The loss is measured with backscatter reflectometry over a wavelength range of 1,528 to 1,608 nm in a 7-m long spiral waveguide. The minimum loss measured is 0.05±0.015 dB m−1near a wavelength of 1,595 nm. The values plotted have been calibrated for spiral curvature using equation (1). A measurement window of 5 nm is applied14,17. Error bars are included on each point and have been computed by standard deviation of three independent measurements. The minimum loss measured is 0.05±0.015 dB m −1 near a wavelength of 1,595 nm. The values plotted have been calibrated for spiral curvature using equation (1). A measurement window of 5 nm is applied [14] , [17] . 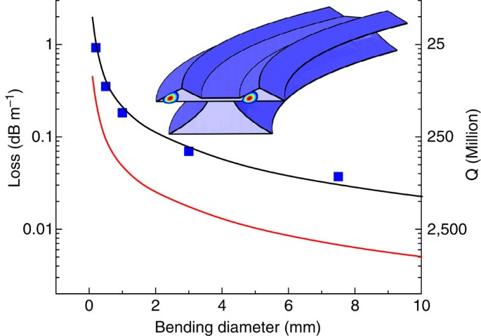Error bars are included on each point and have been computed by standard deviation of three independent measurements. Figure 3: Bending loss data plotted versus the bending diameter. The blue squares are data points obtained from Q measurement on resonators of varying diameters. The black curve is a fit to the data using roughness data provided in the text and obtained using an AFM. The principle source of roughness is the lower interface, and an estimate of the bending loss in case this surface can be smoothed to the level of the upper surface is provided as the red curve. The inset shows a modified version of the spiral design in which a waveguide ridge is created so as to provide both interior and exterior guiding in the spiral. The two colour-graded regions give the mode intensity profile. Full size image Figure 3: Bending loss data plotted versus the bending diameter. The blue squares are data points obtained from Q measurement on resonators of varying diameters. The black curve is a fit to the data using roughness data provided in the text and obtained using an AFM. The principle source of roughness is the lower interface, and an estimate of the bending loss in case this surface can be smoothed to the level of the upper surface is provided as the red curve. The inset shows a modified version of the spiral design in which a waveguide ridge is created so as to provide both interior and exterior guiding in the spiral. The two colour-graded regions give the mode intensity profile. Full size image Backscatter characterization of cascaded-spiral delay lines Figure 2c shows four spirals cascaded on a single wafer to create a 27 m (physical length) waveguide. Each spiral is approximately 4 cm in diameter. The lithography for the spirals involved exposure and stitching of four distinct lithography fields using a Canon FPA 3000 iW stepper tool. The angle-cleaved input facet is in the upper left corner of Fig. 2c . Each spiral features inward and outward, interlaced Archimedean-shaped waveguides that are connected at the spiral centre by an adiabatic coupler. The adiabatic coupler features a completely undercut silica guide that is designed so as to maintain propagation in the fundamental transverse mode through the clockwise to counter-clockwise turn. As shown below, the adiabatic coupler introduces about 0.1 dB insertion loss. In the present design, the constraints imposed on this completely undercut adiabatic coupler when combined with etch non-uniformity over the 9.5 cm×9.5 cm wafer area limits the silicon undercut to about 60 μm. This causes significant interaction of non-fundamental, radial modes with the silicon pillar as noted above. As a result, the backscatter data in Fig. 2d show an apparent increased loss as light propagates through the first two spirals. Moreover, the higher-order modes cause a discontinuity in the backscatter at the large radii, waveguide interconnection between spirals. These conclusions are confirmed through measurements on smaller area, cascaded spiral designs in which a progression of deeper undercuts completely removes the discontinuity and reduces the apparent loss in the entrance spirals. They are also confirmed by the apparent reduction of attenuation in the third and fourth spirals (see Fig. 2d ), wherein we believe propagation is primarily in the fundamental mode as a result of high-order mode filtering provided by spirals one and two as well as their interconnections. It is also significant that the backscatter discontinuity between spirals three and four is weak, also reflecting propagation primarily in the fundamental mode. Analysis of waveguide attenuation in any of the spirals of Fig. 2c is performed by plotting the ratio of out-going to in-going backscatter strength at equidistant points from the spiral centre. Such a plot for spiral 3 is shown in Fig. 4 . The slope of the linear fit gives approximately 0.1 dB m −1 loss for the waveguide, while the intercept gives an insertion loss for the adiabatic coupler of less than 0.1 dB. A similar value is obtained for spiral 4, while spirals 1 and 2 show an apparent waveguide loss of 0.2 dB m −1 , presumably because of the presence of higher-order radial modes. The small difference in optical loss (0.08 versus 0.1 dB m −1 ) for the spirals shown in Fig. 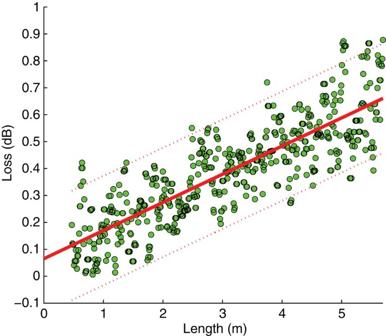2a and c might reflect slight process variation in the fabrication of these devices. Figure 4: Analysis of waveguide loss and adiabatic coupler insertion loss using backscatter data. Green data points are generated by taking the ratio of backscatter signals at symmetrically offset distances away from the adiabatic coupler in spiral 3 ofFig. 2c. The intercept reveals the insertion loss of the coupler as given by a range of possible values falling within a confidence interval. The fitted line (red solid line) slope of about 0.1 dB m−1provides a measure of the waveguide attenuation rate and is in reasonable agreement with the spiral inFig. 2a. The dotted red lines provide the 95% confidence interval. Figure 4: Analysis of waveguide loss and adiabatic coupler insertion loss using backscatter data. Green data points are generated by taking the ratio of backscatter signals at symmetrically offset distances away from the adiabatic coupler in spiral 3 of Fig. 2c . The intercept reveals the insertion loss of the coupler as given by a range of possible values falling within a confidence interval. The fitted line (red solid line) slope of about 0.1 dB m −1 provides a measure of the waveguide attenuation rate and is in reasonable agreement with the spiral in Fig. 2a . The dotted red lines provide the 95% confidence interval. Full size image The adiabatic transition used to connect the clockwise and counter-clockwise Archimedean spirals was designed by applying a variational analysis to the following functional. where κ ( s ) is the curvature of the waveguide and s is the arc-length. Variation of this equation minimizes the adiabaticity condition over the waveguide. By applying the variation to a third-order polynomial subject to boundary conditions of smooth connection up to the first-order derivative of curvature with the Archimedean spiral, a numerical function for the 'S-shape' bend was generated. The S-waveguide width used in the variation was selected so as to allow full undercut of the silica on etching. Loss spectrum and bending loss The backscatter reflectometer measurement is based on a frequency sweep method. By degrading spatial resolution, narrower spectral scans are possible so that spectral variation of the waveguide loss can be measured. In Fig. 5 , spectral data of waveguide loss in a 7-m spiral is presented with the measurement window set to 5 nm (spatial resolution of 200 μm). A minimum value of 0.05±0.015 dB m −1 is measured near 1,595 nm. There is, overall, a weak variation in the apparent loss rate. None of the features seem to be associated with molecular absorption. To obtain the dependence of attenuation on waveguide bending, the Q factor of disk resonators of varying diameters is measured. Optical attenuation as low is 0.037 dB m −1 is attained (see Fig. 3 ), corresponding to an optical Q factor of 670 million. AFM measurement of the upper, wedge and lower surfaces have also been performed on these resonators giving corresponding root mean squared roughness variances of 0.15 and 0.48 nm with correlation length of approximately 200 nm for the upper and wedge surfaces, respectively. The roughness of the lower surface is as large as 1–2 nm in amplitude, but occurs in concentric ring patterns, suggesting that a complex surface interaction takes place during undercut of the silicon. The lower side roughness (assuming a 200 nm correlation length) has been used as a fitting parameter to model the loss versus diameter in Fig. 3 (see Methods for discussion of model). Also, a projection of the predicted loss is given assuming that the lower surface roughness could be reduced to that of the upper oxide surface. In the current design, loss levels lower than 0.01 dB m −1 could be realized. Significantly, the AFM data in conjunction with the optical attenuation data show that thermal oxide is an excellent optical material. Indeed, 0.037 dB m −1 is a loss value that is close to that of the first technologically successful optical fibre [20] . Concerning the stability of this result, based on early work in silica microspheres [21] , it is not expected that water adsorption will impact Q stability for the larger resonator diameters studied here. Indeed, neither resonators nor spiral waveguides experienced any measurable degradation over measurement periods that lasted for several days. Optical buffer demonstration As a simple test of the delay line such as might occur in optical buffering, a 13.5-m double spiral was used to delay a 2.5 Gb s −1 data stream. For this, the light output from an external-cavity semiconductor laser (New Focus, Velocity 6300) was modulated using a lithium niobate modulator (EOspace, intensity modulator AZ-OK5-10) and coupled into the delay line. The delay line was mounted onto a six-axis aligner and the input and output fibres were coupled using precision six-axis aligners. The output was passed through a variable attenuator and detected using a high-speed photo-detector (New Focus, model 1554). Eye patterns of the detected input and output streams were averaged over 10 s with no visible degradation or change in the structure of the eye pattern. In this specific test, the optical delay line stored ~170 bits. At 10 Gb s −1 , it would contain 680 bits. Both the setup and the eye-pattern data are presented in Fig. 6 . 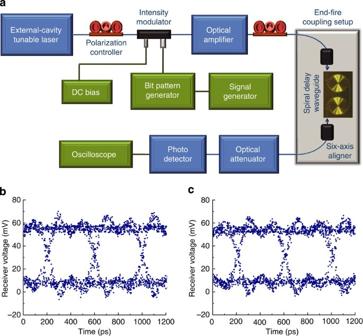Figure 6: Demonstration of the spiral waveguide in the function of data delay as might occur in an optical buffer. (a) Experimental setup used to test a 13.5-m long cascaded spiral in the function of a buffer for a 2.5 Gb s−1data stream. Beginning in the upper left of the panel, a single-frequency laser source is modulated to create a pseudorandom bit stream. The bit stream is amplified and coupled into the spiral delay line. Subsequent to the delay, the signal is attenuated, detected and displayed on an oscilloscope to generate eye patterns. Polarization controllers are also used to launch signals on either the TE or TM mode of the delay line. (b) Eye patterns generated with the 13.5-m spiral delay replaced by a fibre optical cable. (c) Eye patterns generated with the data stream buffered in the 13.5-m spiral delay. The eye patterns of the detected input and output data streams were averaged over 10 s with no visible degradation or change in the structure of the eye pattern. Figure 6: Demonstration of the spiral waveguide in the function of data delay as might occur in an optical buffer. ( a ) Experimental setup used to test a 13.5-m long cascaded spiral in the function of a buffer for a 2.5 Gb s −1 data stream. Beginning in the upper left of the panel, a single-frequency laser source is modulated to create a pseudorandom bit stream. The bit stream is amplified and coupled into the spiral delay line. Subsequent to the delay, the signal is attenuated, detected and displayed on an oscilloscope to generate eye patterns. Polarization controllers are also used to launch signals on either the TE or TM mode of the delay line. ( b ) Eye patterns generated with the 13.5-m spiral delay replaced by a fibre optical cable. ( c ) Eye patterns generated with the data stream buffered in the 13.5-m spiral delay. The eye patterns of the detected input and output data streams were averaged over 10 s with no visible degradation or change in the structure of the eye pattern. Full size image There has been no attempt to reduce footprint in this study, as the emphasis has been on reduction of attenuation rate and demonstration of scalability. However, a modification of the current design is shown in Fig. 3 as an inset. This design uses a ridge geometry produced by a second wet etch to locally confine the mode to both sides of the spiral and leads to a considerable improvement in the area utilization of the wafer. By using the surface roughness measurements described above, we estimate that a comparably low-loss, 100-m long structure could be fabricated in the same footprint as the cascaded spiral in Fig. 2c . Specifically, in the current design ~200 μm per waveguide is used in the Archimedean spiral. In the ridge design, this could be reduced to 70 μm per waveguide. By extension of the stitching method already demonstrated here, it would then be possible to lithographically stitch 10 spiral fields onto an 8 in wafer for a total path length of 250 m. Finally, the integration of this optical delay with an optical circuit is also under study. By using a silicon nitride taper design it is possible to adiabatically and selectively couple a single-mode nitride waveguide to the fundamental mode of the spiral structures described here. This is possible because the fundamental transverse mode of the delay line features the largest effective index (as it has the largest propagation constant β ). As such, a silicon nitride (refractive index 2.0) waveguide taper of thickness ~200 nm can be tapered so as to reduce its effective index to the point of coupling with only the fundamental transverse mode. Using input and output silicon-nitride adiabatic couplers, the delay-line would function essentially as a single transverse mode device, and could be interfaced directly to conventional photonic circuits on silicon. Fabrication of spiral waveguide Waveguides and disks were fabricated on (100) prime grade float zone silicon wafers. The oxide was prepared using the following procedure. An overall 8 μm oxide film was grown by wet oxidation process. Finally, a dry oxidation process was performed for 24 h. The temperature for all the oxidation processes was 1,000 °C. Photo-resist was patterned using a GCA 6300 stepper for disks and Canon FPA 3000 iW stepper for spiral waveguides. Post-exposure bake followed in order to cure the surface roughness of the photo-resist pattern, which acted as an etch mask during immersion in buffered hydrofluoric (HF) solution (Transene, buffer HF improved). The isotropic and uniform etching characteristic of buffered HF solution resulted in oxide disks and waveguides having very smooth wedge profile. The reproducibility of the etch is excellent. Specifically, waveguide width control studies for waveguides on the same wafer show a ±0.25 μm variation in width. After the conventional cleaning process to remove photo-resist and organics, the silicon under the oxide structures was isotropically etched by xenon difluoride to create an air-cladding whispering-gallery waveguide. Buffer patterns were introduced around the waveguide to prevent non-uniform undercut by loading effect during the xenon difluoride etching. Scattering loss modelling In the waveguide, transmission loss results from two sources: the absorptive material losses and scattering loss due to the surface roughness. Through Q versus resonator diameter studies, we conclude that scattering losses are the dominant source of loss in the structures tested ( Fig. 3 ). To model these losses, we adapted a general approach reported elsewhere [9] , [22] , [23] . The rough interface induced radiation loss is calculated via an equivalent volume density, which could be evaluated from the roughness profile and surface electric field where ω is the radial frequency of the light, ε 0 is the free space permittivity, n 0 and n 1 are the refractive index of waveguide and cladding, respectively, and gives the electric field at the interface. From this, the far field radiation as well as the corresponding loss can be evaluated. Assuming that the roughness profiles at top, bottom and sidewall interfaces are mutually uncorrelated, the scattering loss α sc is given by [22] , [23] where is the Poynting vector generated by the equivalent volume density, β is the propagation constant, k 0 is the wave number and is the Fourier transform of the autocorrelation function of the surface roughness profile. Herein, the vectorial electric field at the boundary is calculated using FEM simulation. To determine the surface profile, AFM measurements of the upper, wedge and lower surfaces have also been performed. The roughness profiles are fit to a Gaussian model [22] , [23] , [24] , which yields corresponding root mean squared roughness variances of 0.15 and 0.48 nm with correlation length of approximately 200 nm for the upper and wedge surfaces, respectively. Then, the numerical integration over a spherical surface surrounding the current distribution yields the estimation of the scattering loss. How to cite this article: Lee, H. et al . Ultra-low-loss optical delay line on a silicon chip. Nat. Commun. 3:867 doi: 10.1038/ncomms1876 (2012).